Combinatorial molecular optimization of cement hydrates Despite its ubiquitous presence in the built environment, concrete’s molecular-level properties are only recently being explored using experimental and simulation studies. Increasing societal concerns about concrete’s environmental footprint have provided strong motivation to develop new concrete with greater specific stiffness or strength (for structures with less material). Herein, a combinatorial approach is described to optimize properties of cement hydrates. The method entails screening a computationally generated database of atomic structures of calcium-silicate-hydrate, the binding phase of concrete, against a set of three defect attributes: calcium-to-silicon ratio as compositional index and two correlation distances describing medium-range silicon-oxygen and calcium-oxygen environments. Although structural and mechanical properties correlate well with calcium-to-silicon ratio, the cross-correlation between all three defect attributes reveals an indentation modulus-to-hardness ratio extremum, analogous to identifying optimum network connectivity in glass rheology. We also comment on implications of the present findings for a novel route to optimize the nanoscale mechanical properties of cement hydrate. More than 20 billion tons of concrete produced annually contribute 5–10% to the worldwide anthropogenic carbon dioxide production [1] . One strategy to reduce this environmental footprint is to enhance concrete’s specific stiffness or strength [2] , [3] by optimizing the molecular-level properties of calcium-silicate-hydrates (C-S-H) [4] , [5] , [6] , [7] , [8] , the binding phase of concrete, validated against an array of nano-texture and nanomechanical experiments. In this scheme, a combinatorial database of atomic configurations of C-S-H would be generated by simulation and validated against available structural and mechanical data, with each configuration having a well-defined set of defect attributes as well as a set of corresponding mechanical properties such as elastic modulus and hardness. Optimization then consists of screening the database for the desired properties against the defect attributes, essentially in the spirit of structure–property correlation. The C-S-H binding phase comprises small nanoparticles of 5 nm average diameter [5] , products of reactions between anhydrous calcium silicates and water that form a gel-like network of variable stoichiometry [9] . We have recently reported a model molecular structure of C-S-H, attained through computational simulations that were consistent with experimentally measured average composition, density, scattering and spectroscopic signatures [4] . It is worth mentioning that although Dolado et al. [8] adopted a glass-quenching approach to produce an amorphous structure of C-S-H, we chose to start from the crystalline molecular structure of tobermorite. In fact, at low calcium-to-silicon ratio (C/S), method of Dolado et al. [8] yields a disordered glassy structure for C-S-H, while our approach leads to dominant layered signatures as seen in experiment. In the present work, this model is used to create the database of atomic configurations and corresponding defect attributes and mechanical properties for a wide range of C-S-H chemical compositions. Before using this database to screen for optimum mechanical behaviour, we compare the simulation results to available experiments, consisting of drying measurements, small angle neutron scattering (SANS), inelastic neutron scattering (INS), solid-state nuclear magnetic resonance (NMR) by others and by us, and our own wavelength dispersive spectroscopy, nanoindentation and transmission electron microscopy (TEM) experiments. These comparisons provide model validation and to gain insights into the system-level properties of the ensemble. We are especially interested in the effects on the mechanical behaviour of two types of defects. The first is the C/S ratio, which is well-known in cement chemistry. It can be defined as a measure of points defects (vacancies) in the silicate network [10] . The second type of defect pertains to variations that exist in the medium-range environment of the Si-O and Ca-O networks. It is most simply defined in terms of the first sharp diffraction peak in the Si-O and Ca-O partial structure factor, which is familiar in the study of silica glasses [11] . Effect of C/S ratio on the molecular structure of C-S-H The database for the combinatorial screening of mechanical behaviour is obtained by creating an ensemble of atomic structures of C-S-H with each member characterized by a known value of the C/S ratio over the range of 1.1 to 2.1; all the atomistic models are created consistently according to the procedure explained in Methods section and Supplementary Methods . This is achieved by randomly cutting silica chains (removing a number of charge-neutral SiO 2 groups from 11 Å tobermorite) to increase the C/S ratio, allowing in the course of this procedure an account for reactivity through empirical reactive potentials. In applying combinatorial optimization to better understand the relation between defect attributes and mechanical behaviour of C-S-H hydrates, we search the generated database for atomic configurations that have optimum mechanical properties, and meanwhile we determine the defect attributes specifying these configurations. By mechanical properties, we mean the ratio of indentation elastic modulus (M) to indentation hardness (H). This M/H ratio is distinct from indentation toughness that refers typically to fracture toughness and depends also on indentation crack length [12] ; here, high M/H describes a material of low elastic strain limit. By defect attributes, we consider C/S as an overall measure of chemical composition and two correlation lengths characterizing medium-range environments of Si-O and Ca-O networks. It is not known a priori whether atomic configurations having optimum M/H actually exist, and if so, which defect attributes are relevant. Thus, we begin our screening by first considering only the defect attribute C/S, as the database generated allowed for variations in atomic configurations at fixed values of C/S ( Supplementary Methods ). Although others [4] , [13] , [14] , [15] have calculated elastic properties of distinct mineral phases such as tobermorite polymorphs and jennite via atomistic simulation methods, our approach provides a comprehensive screening of mechanical properties for the C-S-H phase as a function of its chemical composition. Regarding experimental aspects, although correlations between chemical composition and mechanical properties of synthetic C-S-H gels [16] , [17] , [18] , [19] , [20] (fully cured or calcium-leached cement pastes [21] ) have been previously reported, our approach provides a venue to directly assess mechanical properties of the elementary C-S-H nanoparticle as a function of C/S ratio. To be specific about the different defect attributes considered, we show a typical atomic configuration of tobermorite 11 Å (ref. 22 ) in Fig. 1a . The unit cell contains the silica chains ( Fig. 1b ) and Ca atoms in two distinct environments, intralayer Ca ( Fig. 1c ) and interlayer Ca in the interlayer spacing (between adjacent calcium-silicate sheets as highlighted in Fig. 1d ). Hereafter, the intralayer and interlayer calcium atoms are referred to as Ca and Cw, respectively. We introduce two correlation lengths λ and λ ’ (see Fig. 1a ). Here, λ is the medium-range correlation length as measured on Si-O-Si-O motifs and defined for silica glasses [11] , [23] . Similarly, λ ’ is the medium-range correlation length measured on Cw-O-Cw-O motifs. Both λ and λ ’ are present at around 4.3 and 4.6 Å in experimental total radial distribution function, respectively [24] . We will show that each of these two correlation lengths plays a different role in its influence on the mechanical properties, as they pertain to two distinct medium-range order environments in C-S-H atomic structure. 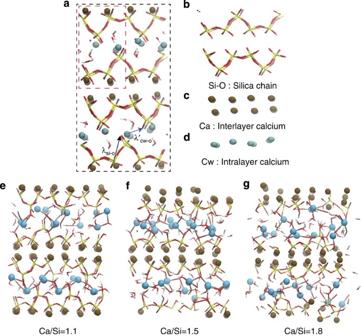Figure 1: Effect of C/S ratio on the molecular structure of C-S-H at the nanoscale. (a) The unit cell of tobermorite 11 Å is enclosed by black dashed line. The brown and cyan spheres represent intra- and interlayer calcium ions, respectively. Red and yellow sticks depict Si-O bonds in silicate tetrahedra. White and red sticks display hydroxyl groups and water molecules. By repetition of unit cells in all lattice vectors, a (2*2*2) supercell of the molecular structure of tobermorite 11 Å is constructed for representation and is outlined by dashed red line. The medium-range correlation lengthsλandλ’, which pertain to Si-O and Cw-O network are represented by dashed black and blue arrows, respectively. The solid skeleton of tobermorite consists of three parts: (b) silica chains, (c) calcium interlayer and (d) calcium intralayer. (e–g) Molecular model of C-S-H at C/S=1.1, 1.5 and 1.8. (e) At C/S=1.1, a lamellar structure is presented with minor defects in silica chains, reminiscent to that of 11 Å tobermorite. The interlayer regions contain counter charge-balancing calcium ions, hydroxyl groups and water molecules. (f) At C/S=1.5, several bridging tetrahedra are removed from the silicate chains. The interlayer calcium ions are still organized in well-defined sites. (g) The C/S ratio is further increased to 1.8 by removal of more silica tetrahedra. This indicates that from low to high C/S ratio, the C-S-H’s molecular structure changes from layered to a more amorphous structure. Figure 1: Effect of C/S ratio on the molecular structure of C-S-H at the nanoscale. ( a ) The unit cell of tobermorite 11 Å is enclosed by black dashed line. The brown and cyan spheres represent intra- and interlayer calcium ions, respectively. Red and yellow sticks depict Si-O bonds in silicate tetrahedra. White and red sticks display hydroxyl groups and water molecules. By repetition of unit cells in all lattice vectors, a (2*2*2) supercell of the molecular structure of tobermorite 11 Å is constructed for representation and is outlined by dashed red line. The medium-range correlation lengths λ and λ ’, which pertain to Si-O and Cw-O network are represented by dashed black and blue arrows, respectively. The solid skeleton of tobermorite consists of three parts: ( b ) silica chains, ( c ) calcium interlayer and ( d ) calcium intralayer. ( e – g ) Molecular model of C-S-H at C/S=1.1, 1.5 and 1.8. ( e ) At C/S=1.1, a lamellar structure is presented with minor defects in silica chains, reminiscent to that of 11 Å tobermorite. The interlayer regions contain counter charge-balancing calcium ions, hydroxyl groups and water molecules. ( f ) At C/S=1.5, several bridging tetrahedra are removed from the silicate chains. The interlayer calcium ions are still organized in well-defined sites. ( g ) The C/S ratio is further increased to 1.8 by removal of more silica tetrahedra. This indicates that from low to high C/S ratio, the C-S-H’s molecular structure changes from layered to a more amorphous structure. Full size image A (3 × 2 × 2) supercell of 11 Å tobermorite is taken as the computational cell used in all the atomistic simulations performed in generating the combinatorial database and in evaluating the structural and mechanical properties to be discussed. Figure 1e–g shows the sensitivity of atomic configurations to variations in C/S ratio in the range of [1.1–1.8]. Keeping in mind our procedure of removing silica groups to increase C/S ratio, we see a progression from a well-ordered lamellar structure at C/S=1.1 to a more disordered structure at C/S=1.8. In particular, the structural surroundings of the interlayer calcium atoms (Cw) as the C/S ratio increases are of prime importance, as this illustrates the subtle effects of introducing vacancies in the silica chains. Effect of C/S on the structure of C-S-H Predicted structural properties of C-S-H at 300 K with C/S ratio are presented in Fig. 2 , and compared directly against experiments. The number of initially absorbed water molecules is predicted to scale linearly with the C/S ratio ( Fig. 2a ), a behaviour that is found in both SANS [5] and drying [25] experiments. There is also consistency with the notion that a removed SiO 2 unit occupies the volume of approximately two H 2 O molecules. As a result of using a reactive force field to model the interactions with absorbed water, a part of the initially grand canonically adsorbed water remains structural molecular water with composition-dependent dynamical anomaly and glassy nature [26] , [27] ( Fig. 2a ), while a considerable amount of water molecules dissociates. The hydroxyl groups predominantly react with interlayer calcium ions to form Ca–OH bonds. The protons bond to non-bridging oxygen of defective silicate chains. To a lesser extent, Ca–OH bonds are also produced by condensation of silica chains, which releases an oxygen atom that combines with H + to form a hydroxyl group. As a consequence of both mechanisms, we find that the number of Ca–OH bonds per Si atom increases linearly with the C/S ratio ( Fig. 2b ), including zero Ca–OH bond for C/S=1, corresponding to 11 Å tobermorite [10] . These predictions are validated by INS data [28] and provide evidence that the present combinatorial simulation approach is able to describe the local water and Ca environments in C-S-H. The level of agreement achieved between simulations and experiments is largely due to the simulated annealing step incorporated in our database generation procedure (see Supplementary Information for further details). 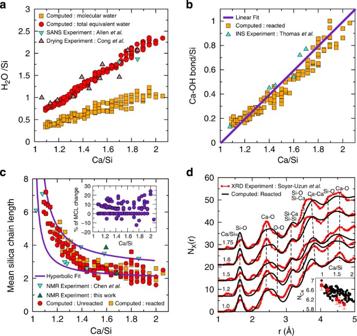Figure 2:Effect of C/S on the nano-texture of C-S-H. (a) The state of water in C-S-H interlayers at 300 K. The total equivalent water contains both the hydroxyl groups and molecular water in the interlayer spacing. The water content is comparable with total equivalent water measured in SANS performed by Allenet al.5and a set of controlled drying experiments done by Cong and Kirkpatrick25. (b) Number of Ca-OH bonds measured via topological analysis at 300 K along with linear fit to the simulation data and their comparison with INS experiments measured by Thomaset al.28(c) The effect of C/S ratio on the mean silicate chain length in reacted and unreacted models at room temperature compared with NMR experiments of this work and those carried out by Chenet al.31and hyperbolic fits to the experimental data. The inset presents the variation of MCL before and after reactive modelling. About 20% of molecular models exhibit extra silica condensation and 5% show silica chains dissociations. (d) The total pair correlation function calculated from molecular dynamics trajectory at 300 K and the comparison with X-ray diffraction experiments of Soyer-Uzunet al.39The inset provides the comparison between coordination number of calcium ion as calculated from atomistic simulation and measured from X-ray diffraction39. This means that the stoichiometry of the solid C-S-H phase can be essentially predicted from atomistic simulation, in the form of: Figure 2: Effect of C/S on the nano-texture of C-S-H . ( a ) The state of water in C-S-H interlayers at 300 K. The total equivalent water contains both the hydroxyl groups and molecular water in the interlayer spacing. The water content is comparable with total equivalent water measured in SANS performed by Allen et al. [5] and a set of controlled drying experiments done by Cong and Kirkpatrick [25] . ( b ) Number of Ca-OH bonds measured via topological analysis at 300 K along with linear fit to the simulation data and their comparison with INS experiments measured by Thomas et al. [28] ( c ) The effect of C/S ratio on the mean silicate chain length in reacted and unreacted models at room temperature compared with NMR experiments of this work and those carried out by Chen et al. [31] and hyperbolic fits to the experimental data. The inset presents the variation of MCL before and after reactive modelling. About 20% of molecular models exhibit extra silica condensation and 5% show silica chains dissociations. ( d ) The total pair correlation function calculated from molecular dynamics trajectory at 300 K and the comparison with X-ray diffraction experiments of Soyer-Uzun et al. [39] The inset provides the comparison between coordination number of calcium ion as calculated from atomistic simulation and measured from X-ray diffraction [39] . Full size image where x is the C/S ratio and a , b , c represent the variability in the nanostructure of C-S-H at a given C/S ratio ( a=b=c =0 corresponds to average pattern for a given C/S ratio and | a |, | b |, | c |<0.2 to only account for polymorphism). The variability in the structure of C-S-H is due to the change in the structure of calcium-silicate backbone at a given C/S ratio. Note that (OH Ca ) and (OH Si ) show hydroxyl groups in calcium-hydroxide and silanol groups, respectively. In Supplementary Discussion , we compare our approach with that of the T/CH model proposed by Richardson [9] , [29] , [30] . We show that our combinatorial approach to C-S-H not only provide a quantitative agreement with experimental data (water content, Ca–OH amount, mean silica chain length and X-ray diffraction pattern) but also has the ability to predict the mechanical properties (elastic modulus and hardness). We term these configurations that share a given C/S composition but differ in atomic level structural details as polymorphs, and later discuss the implications of C-S-H polymorphism. The mean chain length (MCL) of silicates in C-S-H, representative of the degree of polymerization of silicate monomers, is found to decrease nonlinearly with C/S ( Fig. 2c ); there is also a considerable range in the chain length for a set of polymorphs (for example, see C/S=1.8). Although some silicate groups, especially monomers, are found through reactive modelling to condense to form longer chains (see Fig. 2c inset and MCL behaviour in the inset of Fig. 2c ), the amount of monomers at a given C/S before and after condensation reaction varies by <15% ( Supplementary Fig. 3 ). The existence of a range of chain lengths, including monomers, indicated by our simulations is consistent with 29 Si NMR experiments by others [31] and by us, and is the basis of C-S-H polymorphs. Figure 2d compares simulation and experimental synchrotron X-ray data for the total pair correlation function. Both are qualitatively in good agreement; next, simulation data refines the position of all physical correlation peaks in N x ( r ) function for different C/S ratios. However, we note that the Ca–O correlation peak is constantly broader in simulation. This does not affect the calculation of the calcium coordination number that is in quantitative agreement with experiment as shown in the inset of Fig. 2d . We note that the existence of secondary small features in the experimental data that correspond to no identifiable correlation distances and as such can be the results of truncation error in the Fourier transform of the original scattering data. An extensive discussion on the calculation procedure of N x ( r ) is provided in the Supplementary Methods . Effect of C/S ratio on the mechanical properties of C-S-H Several key features can be noted in the experimental validation of model predictions shown in Fig. 3 , wherein the mechanical properties M and H were calculated using a nonreactive potential at 0K (Supplementary Methods). Both simulations and experiments indicate a significant decrease of the average indentation modulus M with increasing C/S ratio ( Fig. 3a,b ). It is not surprising that as C/S increases the calcium-silicate layers become more defective, and as a consequence, mechanical stiffness and anisotropy decrease. A similar trend is found for the hardness H, which is related to the mean pressure sustained beneath the indenter before permanent deformation ( Fig. 3c ). Compared with typical cement hydrates prepared via usual cement dissolution [9] at a median C/S ratio of 1.7, C-S-H prepared at C/S=1 to 1.1 exhibits on average 31% and 48% superior stiffness and hardness, respectively. The C-S-H at low and high C/S ratios responds differently to defect incorporation in the silica chains. To elucidate this particular behaviour, we make use of the calculated full compliance tensor of each numerical sample, and determine the orthotropic in-plane and in-layer elasticity constants, M 1 and M 3 ( Supplementary Methods ) that would be measured in a Hertzian elastic contact loading along orthogonal directions of the calcium-silicate layers [32] . Given the random orientation of C-S-H particles in real cement paste, the experimental assessment of these M 1 and M 3 constants is still out of reach of current indentation technology. Simulation identifies a pronounced anisotropic behaviour of C-S-H at the nanoscale ( Fig. 3b ) in terms of a significant difference between the in-plane stiffness, M 1 , and layer-to-layer stiffness, M 3 . Although both M 1 and M 3 follow the trend of the indentation stiffness M ( Fig. 3a ), we can see that the elastic anisotropy, expressed by the ratio M 1 / M 3 also decreases with increasing C/S ratio. That is, a highly anisotropic C-S-H at low C/S ratios (C/S<1.5) becomes gradually isotropic as long silica chains are shortened on increasing C/S ratio. To further appreciate the impact of texture on properties, it is instructive to employ the isotropic Euclidean norm of C-S-H stiffness tensor, defined as d E ( C iso , C t )=|| C iso − C t || E , where C t and C iso are the full and isotropic parts of the stiffness tensor, respectively [33] . Applied to the C-S-H models, we find that this norm is almost constant for C/S <1.5 ( Fig. 3d ), which correlates well with the observation that C-S-H maintains a tobermoritic layered texture for low C/S ratios (see Fig. 1e–g ). This predominantly lamellar structure is in agreement with experimental observations by TEM [30] , [34] and X-ray diffraction [35] . Indeed, C-S-H at C/S=0.86 shows a lamellar structure ( Fig. 3e ). In turn, for larger C/S ratios, the Euclidean norm decreases ( Fig. 3d ). For such compositions, C-S-H retains some long-range layered texture [36] as TEM images show ( Fig. 3f ), but the increasing amount of defects in the silica chains reduces short-range order ( Supplementary Fig. 3 shows Si-O and Ca-O radial distribution functions characteristic of glassy structures) that decreases elastic anisotropy ( Fig. 3b , M 1 ≈ M 3 ). Furthermore, Bauchy et al. [36] showed that the molecular structure of C-S-H at high C/S ratio (C/S>1.5) is akin to the structure of a model calcio-silicate glass at short range. 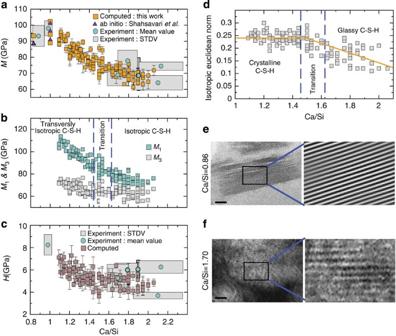Figure 3: Effect of C/S ratio on the mechanical properties of C-S-H at nanoscale. (a) C-S-H solid particle’s indentation modulus, M. The computational data (this work, orange squares) were computed via a nonreactive potential at 0K, and compared with nanoindentation and wavelength dispersive spectroscopy experiments and previous ab initio calculations on 11 and 14 Å Tobermorite19. Gray boxes surrounding experimental mean values indicate standard deviation (STDV) calculated from standard errors by noting that M and Ca/Si are normally distributed (seeSupplementary Methods). (b) Indentation modulus parallel (M1) and perpendicular (M3) to the calcium-silicate layers. (c) C-S-H solid particle's hardness, H. The computed data (brown squares) are compared with experimental values following the same convention as ina. (d) Computed isotropic Euclidean norm as an indication of the level of anisotropy in C-S-H. Orange lines are guide for the eyes. (e) TEM image of C-S-H at C/S=0.8634. (f) TEM image of C-S-H at C/S=1.7 produced from hydration of C3S. In both (e) and (f), TEM imaging conditions were in vacuum at 10−6torr; the scale bar is 10nm. The error bars in atomistic simulations are calculated via computing M or H for multiple configurations along the equilibration trajectory that generated the C-S-H structures for each polymorph. For the sake of clarity,Fig. 3cshows one fewer experimental data point at C/S~1 and H~12 GPa, listed inSupplementary Table 6. Figure 3: Effect of C/S ratio on the mechanical properties of C-S-H at nanoscale. ( a ) C-S-H solid particle’s indentation modulus, M. The computational data (this work, orange squares) were computed via a nonreactive potential at 0K, and compared with nanoindentation and wavelength dispersive spectroscopy experiments and previous ab initio calculations on 11 and 14 Å Tobermorite [19] . Gray boxes surrounding experimental mean values indicate standard deviation (STDV) calculated from standard errors by noting that M and Ca/Si are normally distributed (see Supplementary Methods ). ( b ) Indentation modulus parallel ( M 1 ) and perpendicular ( M 3 ) to the calcium-silicate layers. ( c ) C-S-H solid particle's hardness, H. The computed data (brown squares) are compared with experimental values following the same convention as in a . ( d ) Computed isotropic Euclidean norm as an indication of the level of anisotropy in C-S-H. Orange lines are guide for the eyes. ( e ) TEM image of C-S-H at C/S=0.8634. ( f ) TEM image of C-S-H at C/S=1.7 produced from hydration of C 3 S. In both ( e ) and ( f ), TEM imaging conditions were in vacuum at 10 −6 torr; the scale bar is 10nm. The error bars in atomistic simulations are calculated via computing M or H for multiple configurations along the equilibration trajectory that generated the C-S-H structures for each polymorph. For the sake of clarity, Fig. 3c shows one fewer experimental data point at C/S~1 and H~12 GPa, listed in Supplementary Table 6 . Full size image Understanding maximum M/H via dual-defect framework The goal of our combinatorial optimization is to find atomic configurations that give maximum M/H and correlate those molecular structures with corresponding defect attributes. The correlation of M/H with C/S ratio is shown in Fig. 4 . Notably, some C-S-H configurations, with C/S ratio close to 1.5, exhibit maximum M/H. Next, we consider the thermodynamics stability of these polymorphs to consider their relative prevalence in experimentally accessible C-S-H. 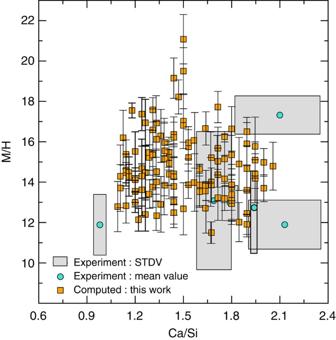Figure 4: M/H as a function of C/S ratio. The simulation results were computed with a non-reactive potential at 0K, and are compared against experimental data. Experimental M/H are shown as mean (points) and uncertainty (gray boxes) calculated by assuming M and H are normally distributed independent quantities that are each characterized by a standard deviation. SeeSupplementary Methods. For the sake of clarity, this graph shows one fewer experimental data point than inFig. 3a, at C/S~1 with M/H~8; seeSupplementary Table 6. Figure 4: M/H as a function of C/S ratio. The simulation results were computed with a non-reactive potential at 0K, and are compared against experimental data. Experimental M/H are shown as mean (points) and uncertainty (gray boxes) calculated by assuming M and H are normally distributed independent quantities that are each characterized by a standard deviation. See Supplementary Methods . For the sake of clarity, this graph shows one fewer experimental data point than in Fig. 3a , at C/S~1 with M/H~8; see Supplementary Table 6 . Full size image Numerous compelling experimental results from this and other experimental studies [5] , [31] confirm our conjecture that C-S-H at the nanoscale can exist in different molecular structures for the same oxide composition, that is, same C/S ratio. Specifically, results from NMR experiments [31] suggest that C-S-H at a given composition can have different MCL, and results from neutron scattering experiments [5] imply that C-S-H of a given composition can exhibit varying water content. Figure 3 shows that calculated indentation modulus and hardness exhibit a range of possible values at a fixed oxide composition for a given C/S ratio. Experimentally measured M and H (for example, C/S~2.1 in Fig. 3a,c ) confirm this potential variation in stiffness and hardness for fixed oxide chemistry. Yet, the existence of polymorphism calls for thermodynamics arguments to assess the co-existence of C-S-Hs of different molecular structure at equilibrium for a given composition. This is achieved in our simulation through the calculation of the free energy of the C-S-H models considerably below their melting point via lattice harmonic approximation theory from the phonon density of state. Interestingly, the free energy content of C-S-H polymorphs is almost constant at a given C/S ratio ( Supplementary Methods ). That similar level of energetic favorability implies that all polymorphs of a given C/S ratio are equi-probable at equilibrium, and thus thermodynamically competitive. This means that a targeted mechanical property at constant C/S ratio cannot be achieved through equilibrium conditions, but relies on the kinetics of silica polymerization and associated disorder assimilation. To consider whether the short-range structural characteristics could explain why M/H is high at a specific C/S ratio, we performed a comprehensive search for correlations among structural characteristics (bond lengths, bond angles and coordination numbers) and mechanical properties. No such short-range correlations were identified. It was these findings that motivated us to consider medium-range correlation lengths as possible defect attributes as captured by the first sharp diffraction peak (FSDP) in covalent glasses [11] , [23] , which captures spatial correlations in the medium-range order ( Supplementary Methods ). Although its origin in amorphous silicate solids is not yet fully understood, it is commonly accepted that the FSDP relates to the periodicity of the boundaries between small adjacent structural cages of SiO 4 tetrahedra [37] . The associated correlation distance in real space is given by λ =7.7/ Q FSDP , where Q FSDP is the position of the FSDP in the partial Si-O structure factor, and the constant 7.7 is the location of the first maximum of the spherical Bessel function J 0 (ref. 38 ). Overall, this distance characterizes how well SiO 4 tetrahedra are packed as it corresponds to the distance between Si atoms and their second coordination shell of oxygen atoms [24] , [39] . Recently, it has been pointed out that as a coarse-grained defect attribute of network glasses, λ plays a significant role in enabling structural characteristics to be correlated with transport and rigidity properties [38] . Moreover, the lack of covalent bonding and the screening effect of structural water molecules make the chemical environment surrounding interlayer calcium atoms susceptible to deformation. This leads to the localization of the deformation at the interlayer region on application of uniform strain field [4] , [40] . This further motivated us to define, in a similar manner, the medium-range correlation length λ ’ in the interlayer calcium environment pertaining to the Cw-O network (see Fig. 1a ). Given the fact that these structural defect attributes, (C/S, λ , λ ’) may not be independent, it is reasonable to ask whether a broader search by screening two or more defect attributes together could be useful. In fact, we may benefit by extending the screening to correlations of M/H against C/S, λ and λ ’. For this purpose, contour plots of M/H values on surfaces of two defect attributes were considered. 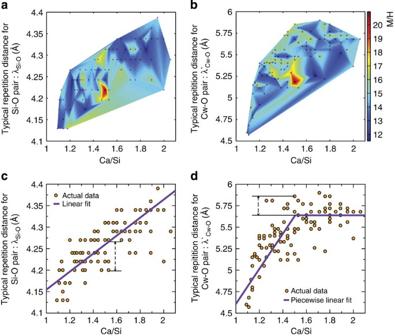Figure 5: Exploring the M/H extremum via the dual-defect framework computed from atomistic simulations. (a) C/S-λ(Si-O) and (b) C/S-λ’(Cw-O). Both contour plots show a region in which M/H is maximized. The correlation among defect attributes (c) C/S-λ(Si-O) and (d)λ’(Cw-O), and their (c) linear and (d) piecewise linear fit to the simulation results, which correlate with highest values of M/H described by packing of silica chains (responsible for higher stiffness) and openness of Cw-O network (responsible for lower hardness). The arrows in (c) and (d) indicate that the samples at Ca/Si~1.5 with high M/H would have lowest Si-O and highest Cw-O medium-range correlation lengths. Figure 5a,b shows the contour plots (colour coded) of M/H on the surface of [C/S, λ ] ( Fig. 5a ) and [C/S, λ ’] ( Fig. 5b ). In both cases, local regions of peak values are clearly identified. According to Fig. 5a,b , two optimum sets of defect attributes exist, one involving (C/S, λ ) and the other (C/S, λ ’), which signifies that optimization of M/H can be achieved through the synergistic sensitivity to two sets of dual-defect attributes. Figure 5: Exploring the M/H extremum via the dual-defect framework computed from atomistic simulations. ( a ) C/S- λ (Si-O) and ( b ) C/S- λ ’(Cw-O). Both contour plots show a region in which M/H is maximized. The correlation among defect attributes ( c ) C/S- λ (Si-O) and ( d ) λ ’(Cw-O), and their ( c ) linear and ( d ) piecewise linear fit to the simulation results, which correlate with highest values of M/H described by packing of silica chains (responsible for higher stiffness) and openness of Cw-O network (responsible for lower hardness). The arrows in ( c ) and ( d ) indicate that the samples at Ca/Si~1.5 with high M/H would have lowest Si-O and highest Cw-O medium-range correlation lengths. Full size image The notion of distributed (synergistic) sensitivity can be examined by correlating the defect attributes, specifically the relations between λ and C/S, and λ ’ and C/S, which are shown in Fig. 5c,d . Within the considerable scatter in the data, it appears that λ increases essentially linearly with increasing C/S ( Fig. 5c ), while λ ’ increases then plateaus ( Fig. 5d ). The increase in λ with C/S ratio corresponds to an increase in the magnitude of tetrahedron–tetrahedron relaxation in the silica chains—which is spatially distinct from the amount of nanometric SiO 2 vacancy defects that correlates with C/S. Although the range of variation of λ is rather small [4.1–4.4 Å], our results are nevertheless in agreement with recent diffraction studies [34] , which show that λ corresponding to Si-O peak in the total diffraction pattern (obtained after Fourier transforming the total X-ray scattering signal) does shift to larger distance on increasing C/S ratio (see Fig. 6 in ref. 12 ). This indicates that for a fixed C/S, the low-lying λ points correspond to atomic configurations where the local environment of the silica chains are more compact, and they therefore contribute to higher stiffness (M). Indeed, configurations of greatest M in Fig. 3a at a fixed C/S=1.5 were those that also exhibit lowest λ . Furthermore, in Fig. 5d , we see that λ ’ reaches its maximum value signalled by a plateau at C/S>1.5. This corresponds to configurations with relatively open Cw-O medium-range environment, which indicates there is more space for deformation. This explains the hardness plateau in Fig. 3c , for relatively stable and low H for C/S>1.5. The appearance of M/H extremum in Fig. 5a,b results from a coupled optimization of λ and λ ’ at C/S=1.5. Therefore, the C-S-H with maximum M/H value is a C-S-H at C/S=1.5, which simultaneously has a minimum in λ and maximum in λ ’. However, it should be kept in mind that these two are correlated. Another way to infer the significance of the peak region of M/H is to interpret M/H as proportional to the inverse of an effective yield strain. To our knowledge, the simultaneous screening of mechanical properties against two defect attributes has not been previously considered in the cement science and chemistry literature. By comparing Fig. 5a,b and Fig. 5c,d , we believe this new approach has broad implications regarding property optimization. Simply stated, in Fig. 4 one seeks an extremum in a single-variable function M/H= f (C/S), whereas in Fig. 5 one seeks a function of two variables, M/H= f (C/S, λ ). Any effects of correlation between C/S and λ would be missed in Fig. 4 . Moreover, the results of Fig. 4 and Fig. 5 suggest that M/H is a property distributed in two defect attributes rather than being fully characterized by the single C/S chemical attribute. This is perhaps to be expected, given the complexity of the molecular structure C-S-H. It is therefore rather gratifying that other structural attributes, the packing of the silica tetrahedra and the medium-range environment of the interlayer Cw-O network, can also affect the mechanical response. This work has benefitted from studies of network-forming glasses [38] , [41] , [42] , which have given further insights into the concept of atom-averaged covalent coordination number, < n >, as a structural attribute capable of identifying optimum network connectivity [43] , [44] . From measurements of microhardness, peak values of indentation fracture toughness on binary Ge-Se glasses were found when the properties were screened against < n > (ref. 41 ), similar in spirit to our screening against medium-range correlation lengths (in addition to chemical composition C/S) in Fig. 5 . Recently, it was pointed out that the defect attribute associated with the first sharp diffraction peak (see Introduction) plays a fundamental role in revealing extremum or anomalous behaviour in rigidity deformation and transport properties of network glasses [38] . Here again we see a connection with the present findings: a relation can be established between system-level properties and defect attributes in both network glasses, and in C-S-H. In this work, we introduce an approach of combinatorial screening of indentation stiffness and hardness for realistic models of cement hydrates against a set of structural defect attributes. We find peak values in the measured M/H in two defect-attribute sets, (C/S, λ ) and (C/S, λ ’). Based on considerations of various cross correlations among the defect attributes, we conclude M/H is a distributed property in that the relevant attributes of the underlying atomic configurations are coupled. We interpret the nature of the correlation to lie in the connectivity of medium-range environments, such as packing of silica network and openness of Cw-O regions of the cement hydrates. These medium-range structural attributes explain the observed mechanical properties: for a range of C/S, closer silica chain packing increases C-S-H stiffness, and larger distances between Cw-O pairs facilitates deformation and lowers hardness until a saturation of this effect at C/S~1.5. For a fixed C/S such as 1.5, polymorphs with closer packing of silicate tetrahedra exhibit higher stiffness, and those that also have increased distance between these calcium-oxygen sites exhibit lower hardness. Moreover, we believe the defect-attribute coupling to be a manifestation of inorganic molecular networks that may also describe other multi-component systems with structural complexities across the nano- and mesoscale. For future studies, it would be appropriate to focus on the characterization of pores and confined water in cement hydrates, and to assess meso-, micro- and macroscale toughness of concrete at the large scale. To achieve this, new mesoscale models [45] , [46] have to be developed and validated, and appropriate databases generated. These will involve additional defect attributes such as particle packing density, pore size distribution and connectivity, and the effects of water in various spatial confinements [47] , [48] , [49] , [50] . The combinatorial approach introduced here is anticipated to aid those efforts, and may contribute to optimized concrete design that has the potential to ultimately reduce material consumption and associated CO 2 production. Indeed, although the CO 2 emission of cement clinker production scales with the volume of the concrete structural elements (beams, columns, etc), the structural strength scales with their cross-sectional area. By adopting a limit state design approach, it is thus expected that an increase of the macroscopic concrete material strength by a factor of δ allows reducing the environmental footprint to δ −1 for pure compressive members such as columns and shells, δ −2/3 for beams and δ −1/2 for plates [3] . As contemporary concretes are characterized, on average, by high C/S ratios, an increase in C-S-H strength achieved by reducing C/S from 1.7 to 1.1 (for instance with silica flour additions and proper curing conditions) can entail a reduction of material volume and associated CO 2 emissions for compressive members. This projection assumes that the enhanced stiffness or hardness achieved by controlling molecular-level structures of C-S-H nanoparticles can be translated directly to the large-scale behaviour of concrete, and that hardness correlates directly with compressive strength (see Supplementary Methods ). Specifically, further investigations are necessary to understand how molecular and mesoscale features and associated properties influence the structure and properties of networks or grains of calcium-silicate-hydrates, understand the effects of particle shape, size and interparticle cohesion, and also which nanoscale properties maximize certain macroscopic properties of concrete—a composite of multiple material phases. Generating the C-S-H database The database for the combinatorial screening of mechanical behaviour is obtained by creating an ensemble of atomic structures of C-S-H with each member characterized by a known value of the calcium to silica ratio, C/S, lying in the range [1.1, 2.1]. The procedure used to generate this ensemble consists of seven steps of atomistic-scale simulations, which we summarize here ( Supplementary Figs 1–8 and Supplementary Methods ). First, a supercell of the atomic structure of tobermorite 11 Å according to Hamid [22] is constructed. With the silicate chains having no defects, there are no hydroxyl groups in the system at this stage. Moreover, the chains are infinite in extent. Next, all water molecules are removed from the interlayer spacing in the supercell. In step three, 150 samples are prepared by randomly cutting the silica chains (removing a number of charge neutral SiO 2 groups). Each removal causes the C/S ratio to increase. By cutting the chain at different locations, several samples with the same C/S ratio are thus generated. In this step, the interlayer calcium atoms are first allowed to relax by energy minimization using CSH-FF potential [52] ( Supplementary Material Tables 1–4 ), followed by all the other atoms and the supercell dimensions. In step four, water molecules are introduced back using a Grand Canonical Monte Carlo method using the same potential, simulating equilibrium with bulk water at room temperature. At step five, the inserted water molecules are allowed to react with the interlayer calcium and the silica groups by running semi-classical molecular dynamics simulations using the ReaxFF potential [7] . To accelerate the reaction, the system temperature is raised to 500 K, which is well below the melting point of C-S-H. At this stage, the results show that some of the interlayer water molecules dissociate to hydroxyl groups and protons. Minor condensations/dissociation of silica chains are also observed in some samples. Of the 150 samples generated, all were amenable to equilibration within ReaxFF over the finite trajectory duration. In step six, a comprehensive topological analysis is performed to identify the local environment of species, in the process of distinguishing between different types of oxygen, hydrogen and calcium atoms. This facilitates the transition from the use of ReaxFF to the non-reactive potential, CSH-FF, which is well suited to study the mechanical properties of C-S-H phases and used for that purpose [52] . In the final step, a 3-ns-long simulated annealing is performed on each sample to bring the temperature from 500 to 300 K at ambient pressure, using the CSH-FF potential. The annealing procedure consists of 1 ns simulation at 500 K followed by a 1-ns ramp to decrease the temperature to 300 K and additional 1 ns at 300 K for relaxation. All the chemical and structural characterizations along with the mechanical properties (indentation modulus and hardness) are calculated from the atomic configurations prepared by this procedure. Calculation of mechanical properties in atomistic simulation It is the central goal of this work to probe the relation between mechanical properties (stiffness and hardness) and the various defect attributes via a combinatorial database established by atomistic simulations. To exclude the rate effect in the calculation of mechanical properties in molecular dynamics simulation, such calculations are performed via the energy minimization technique at 0 K. Recently, Carrier et al. [53] reported negligible difference between the elastic properties obtained via finite temperature calculations using elastic bath technique and those measured by energy minimization method for low water-containing clays. We are interested in the average elastic properties of the C-S-H solid particles expressed in terms of the indentation modulus (M), which is determined from the full compliance tensor of each C-S-H model, and evaluated by M=4 G (3 K + G )/(3 K +4 G ), where G and K are Voigt–Reuss–Hill shear and bulk moduli, respectively ( Supplementary Methods ). In our atomistic simulations, hardness (H) was determined by using the Mohr–Coulomb failure criterion, applicable to cohesive-frictional materials such as C-S-H [54] . This is achieved through a coupled biaxial (shear-compressive) deformation scheme in several independent deformation paths similar to those used for studying validity of the Cauchy–Born rule [55] , [56] , [57] , [58] . The hardness is calculated from friction angle ( ϕ ) and cohesion ( c ) ( Supplementary Methods ). Both indentation modulus and hardness are averaged among those configurations obtained from several statistically independent time frames along the equilibrium molecular dynamics (MD) trajectory for each polymorph. Experimental analysis To provide experimental validation of the predicted changes in C-S-H stiffness and hardness with chemical composition, we synthesized common industrial cement pastes under varying conditions ( Supplementary Tables 5 and 6 and Supplementary Method ). We implemented a statistical chemomechanical clustering method of composition, indentation modulus and hardness at the sub-micrometre scale ( Supplementary Figs 9–13 and Supplementary Method ). The Ca/Si ratio for each cement paste was determined by clustering X-ray wavelength dispersive spectroscopy data comprising 400 nanoscale volumes (voxels) per sample. The indentation modulus and hardness were quantified at similar length scales, via clustering analysis of nanoindentation grids [54] , [59] , [60] , [61] including 400 voxels per sample. The mechanical properties thus obtained were corrected for the effect of mesoscale porosity to arrive at the indentation modulus and hardness of the monolithic or solid C-S-H nanoparticle [21] , [62] , for direct comparison with the simulation data. In addition, 1 H- 29 Si cross polarization magic angle spinning NMR spectroscopy was employed to confirm silicate chain length, and TEM was conducted in vaccuo to visualize the C-S-H structure. How to cite this article: Qomi, M. J. A. et al. Combinatorial molecular optimization of cement hydrates. Nat. Commun. 5:4960 doi: 10.1038/ncomms5960 (2014).